Selective chemical protein modification Modification of proteins is widespread throughout nature, increasing the diversity of protein structure and hence function by up to two orders of magnitude [1] . Yet, our ability to synthetically mimic nature’s capacity to install such modifications is essentially limited by the chemistry that is available. Reaction at a single amino acid or site, among a sea of reactive carboxylic acids, amides, amines, alcohols and thiols, is a significant and exciting challenge in both chemo- and regioselectivity. Potential transformations, if they are to be relevant, are moulded by the need for biologically ambient conditions (that is, <37 °C, pH 6–8, aqueous solvent) so as not to disrupt protein architecture and/or function. Ideally, this should proceed with near total conversion to generate homogenous constructs [2] , [3] , [4] . The applications of modified proteins are many; they are as varied as the in vivo tracking of protein–fluorophore conjugates [5] to the polyethylene glycol (PEG)ylation of therapeutic proteins to reduce immunogenicity [6] , from the production of materials with novel properties [7] to probing the mechanism of pathological enzymes [8] . While many past examples of so-called ‘bioconjugation’ exist (and even dedicated journals), those that teach a strong strategic lesson are more rare. The rigour of the chemical approach (including proper characterization) has been lacking—supplanted perhaps by a pragmatic desire for useful product. In an era now hungry for precise molecular knowledge of protein function, previously rare (historical) examples of precise protein chemistry become vital. We (subjectively) consider that a seminal example can be found in the work of Wilchek [9] and later Bender [10] and Koshland [11] . Their chemical conversions of serine to cysteine have, as singularly early examples of site-directed protein mutagenesis, we believe, still not been fully appreciated. It set the stage for approaches that are only now coming to fruition in a broadly applied manner. In a post-genomic era that is more conversant with limitations of ‘gene-only’ methods, this will likely prove uniquely powerful [12] . Over the past two decades, a number of methodologies have emerged (for example, Fig. 1 ) for undertaking modification at both natural and non-standard amino-acid residues, in vitro and in vivo , building on a previously limited toolkit for modification primarily at cysteine and lysine [13] . In this review, we will focus on these key developments that have greatly expanded the protein chemistry reaction palette. In particular, we will highlight merits and current limitations of reactions, in the context of the protein-conjugate bond-type formed. 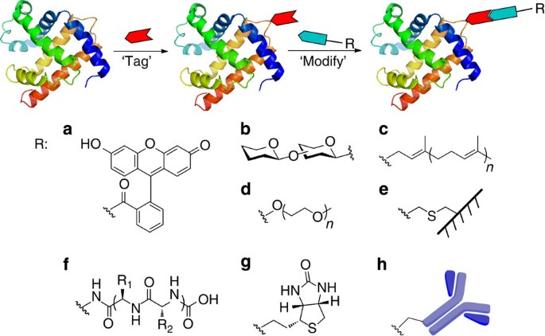Figure 1: A ‘tag-and-modify’ approach to protein modification. A uniquely reactive amino-acid ‘tag’171is installed on a protein surface for reaction with a desired ‘modification’. Examples include (a) fluorophores5,125(b) glycosylation35(c) prenylation37(d) PEGylation87(e) attachment to solid surfaces172(f) peptides44(g) biotinylation90and (h) antibody conjugation159. Figure 1: A ‘tag-and-modify’ approach to protein modification. A uniquely reactive amino-acid ‘tag’ [171] is installed on a protein surface for reaction with a desired ‘modification’. Examples include ( a ) fluorophores [5] , [125] ( b ) glycosylation [35] ( c ) prenylation [37] ( d ) PEGylation [87] ( e ) attachment to solid surfaces [172] ( f ) peptides [44] ( g ) biotinylation [90] and ( h ) antibody conjugation [159] . Full size image Natural amino acids bring with them immediate accessibility without the need for more specialist techniques. Yet, the palette of functional groups is more limited and abundance may play a critical role in determining selectivity and hence precision. Low abundance (for example, cysteine) may allow (re)positioning to allow use of site-selective strategies; this is effective reassignment of the associated codons to encode the site of reaction for a complete and a hence precise alteration. Yet with high abundance, full reaction of all may be unlikely and hence reactions of all may generate (often statistical) mixtures of many products. Moreover, many of the functional groups in proteins are nucleophiles. This creates both a limitation on their use alone (differentiation based on selectivity may be more difficult) and an opportunity (unnatural amino acids (UAAs), see below, may then be designed with very different properties that are chemically distinguishable from this natural nucleophilic set). Cysteine S protein –C bonds As the most robustly nucleophilic of the 20 canonical amino acids, the thiol of cysteine offers a unique reactive handle within proteins, a property exploited extensively in nature [1] . Although pH may need to be controlled, selective reaction at cysteine over other nucleophilic residues such as lysine and histidine can be achieved [14] , while the low abundance (<2%) of cysteine in proteins often allows for facile modification at a single site [3] . In addition to functionalization of a protein of interest, this can also allow ready mutational repositioning and codon reassignment (through Cys→Ser/Gly mutation) [15] . The selective reactions of cysteine with electrophiles such as α-halocarbonyls and maleimides have been suggested for almost a century ( Fig. 2b,c ) [16] . Indeed, iodoacetamide is used routinely for capping before digestion for protein sequencing [17] . Notably, some derivatives react with N-nucleophiles [18] . However, commercial availability and ease of use and synthesis of maleimide derivatives [13] , [19] have led to widespread use (for example, vaccine candidates [20] or modified enzymes [21] ) [13] . Their use results in a reaction typically considered irreversible, yet it has been suggested that this can be reversed by competitive thiols [22] . Hydrolysis of the maleimide adduct moiety can also lead to subsequent decomposition of protein conjugates [22] , [23] ; interestingly, this may advantageously reduce cited reversibility [22] . Thus, potential degradation may be an important consideration, particularly when instability may give rise to an unwanted mixture of products. Interestingly, use of bromomaleimides has opened up the possibility of reversible conjugation, allowing modulation of activity and in vivo monitoring, while also allowing the bridging and stabilisation of native disulfides [19] , [24] . The rare 21st amino acid, selenocysteine, can also be engineered into proteins and used to react with maleimides; greater Se nucleophilicity can allow conjugation selectivity over cysteine residues [25] . 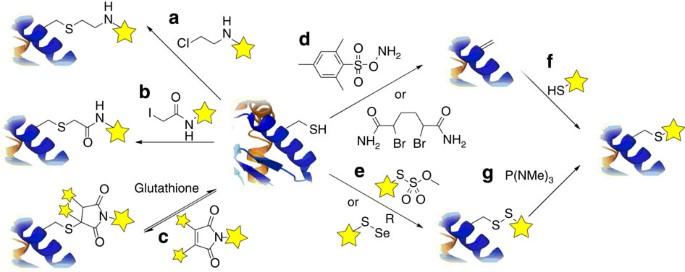Figure 2: Chemical modifications at cysteine. (a) Aminoethylation26,27(b) iodoacetamides17(c) maleimides19,173(d) Dha formation166(e) disulfide formation35(f) reaction of Dha with thiols167and (g) desulfurization of disulfides. Figure 2: Chemical modifications at cysteine. ( a ) Aminoethylation [26] , [27] ( b ) iodoacetamides [17] ( c ) maleimides [19] , [173] ( d ) Dha formation [166] ( e ) disulfide formation [35] ( f ) reaction of Dha with thiols [167] and ( g ) desulfurization of disulfides. Full size image Recently, aminoethylating agents have been used; the resulting thioether products (‘thia-lysines’) can mimic lysines bearing post-translational modifications (PTMs) such as methylation and acetylation, modifications with key roles in eukaryotic cells, particularly in the histone proteins that package DNA ( Fig. 2a ) [26] , [27] . More recently, transition metal-catalysed modifications of cysteine have been reported, such as rhodium-catalysed reaction with diazo compounds, although potential side reactions with tryptophan have been noted as a limitation [28] . Thiyl radicals at Cys can also be utilized for unique chemistries (see Box 1 ). The use of cysteine nucleophiles has traditionally been limited to in vitro application due to the concentration of free thiols in cells (for example, glutathione). Some attempts have been made to conduct selective cellular labelling through introduction of Cys at particularly reactive sites of cell-surface proteins [29] . Box 1: Miscellaneous reactions with utility. While less common, other miscellaneous but nonetheless illustrative reactions exist for modifying both natural and unnatural amino acids in a site-selective fashion. Some rely on differential accessibility to generate selectivity, or utilize specialist reactivities making them less applicable to the general synthesis of proteins, yet they remain useful in certain situations. Among the natural amino acids, tyrosine possesses unique reactivity due to its phenolic hydroxyl group [174] . As a largely nonpolar residue, it is often buried within protein structures, which has led the group of Francis to develop a number of reactions that may modify a surface-exposed tyrosine. These include reactions that modify tyrosine primarily in the ortho -position, such as the use of diazonium salts for diazoarylation [175] , a three-component Mannich-type reaction with a suitable aldehyde and aniline [176] or the oxidative coupling of dialkylanilines in the presence of cerium(IV)ammonium nitrate (CAN) [174] . Alternatively, the hydroxyl group may be alkylated via palladium-mediated π–allyl chemistry [177] . Barluenga’s reagent can introduce an ortho -iodide on tyrosine, although side reactions with other amino acids can occur and must be controlled by careful choice of stoichiometry and pH [178] . These reactions have found use in the modification of viral capsids for materials, pharmaceutical and imaging applications, and have the benefit of using native protein structures [7] . However, such reactions are also often limited to cases where a single exposed tyrosine is present and careful control of reaction site can be undertaken, limiting their more widespread use. A related reaction also discovered by the group of Francis utilizes the aniline analogue of tyrosine to undertake oxidative coupling with aryl-diamines, in a reaction analogous to CAN-mediated coupling of tyrosine [179] . In this latter case, the use of the genetically encoded UAA p -aminophenylalanine allowed a higher degree of site selectivity, even in the presence of tyrosine residues, giving selective conjugation of targeting species to the surface of viral capsids [180] , [181] . These tyrosine and tyrosine-analogue reactions therefore illustrate again how the combination of correct tag and reaction may greatly increase selectivity and efficiency. Recent developments have allowed use of radical and photoconjugations for protein modification. Wittrock et al . [182] first reported the use of the classical radical thiol–ene (thiyl–ene) reaction between thiols and olefins as a method for modifying thiol-containing proteins under ultraviolet irradiation. This has subsequently been exploited at both genetically encoded alkenes [169] , [183] and native cysteine residues [184] to generate glycoprotein mimics [169] , [184] , and for surface immobilisation of proteins [172] . A related reaction, the thiol–yne reaction with alkynes, has also been reported [100] , [185] . Photocrosslinking residues in proteins that exploit the chemistry of photogenerated reactive intermediates have also seen a resurgence. Although the inherent principles for such protein affinity labeling are in fact long-standing [186] , codon reassignment has recently allowed benzophenones [187] , azides [188] and diazirines [189] , [190] to be precisely placed in proteins. While crosslinking is often nonspecific in its target, this method has generated detailed information regarding protein–protein interactions, as well as the binding of small molecules at active and allosteric sites. When combined with proteomic methods, it provides a powerful tool for the elucidation of putative protein-mediated mechanisms, even in complex systems. Cysteine S protein –S bonds The ability of sulfur to alter oxidation state is often exploited in natural redox reactions. Sulfur–sulfur bonds are key in maintaining protein tertiary and quarternary structure via interchain bridges. This property of sulfur can be exploited in the synthetic modification of proteins; formation of disulfides between thiol and cysteine can occur under an ambient atmosphere ( Fig. 2e ). However, rate of reaction is often slow, and disulfide exchange (ideally with kinetic control) is a favoured method for installing modifications; Ellman’s reagent has long been used to quantify free thiols. Additional thermodynamic driving force can be exploited to favour formation of disulfide on-protein but can be unpredictable. Thus, reagents that allow kinetic control have been developed, typically relying upon thiol-specific electrophilicity. The use of methanethiosulfonates and phenylthiosulfonates has allowed quantitative, selective modification of proteins, giving labelled proteins [30] , modified enzymes [31] and glycoconjugates [32] , [33] , [34] . van Kasteren et al . [35] utilized such reagents to generate a mimic of P-selectin glycoprotein ligand-1, via a dual modification with a methanethiosulfonate (to generate a sulfotyrosine mimic) and triazole-forming reaction (to install a mimic of sugar sialyl-Lewis x ). Selenenyl–sulfides show enhanced reactivity ( Fig. 2e ); S–Se intermediates can either be installed on-protein, allowing reaction with the desired thiol (electrophilic strategy), or via addition of a selenenyl–sulfide reagent to cysteine directly (nucleophilic strategy) [36] , [37] . Mechanistically, both routes appear to exploit electrophilic sulfur in the S–Se bond as a source of their chemoselectivity. Lysine and N-terminus N protein –C bonds Despite high natural abundance, lysine remains a popular choice for modification due to the number of successful reactions that can be applied to highly nucleophilic primary amines [4] . This is particularly the case where selectivity (as opposed to reactivity) for the site of modification is perceived not to be important, or where multiple conjugations are desired, for example, in the display of multiple antigens for creation of conjugates as putative vaccines [38] . Preferential conjugation with amines, over the nucleophilic thiol of cysteine, can, in principle, be achieved through use of ‘harder’ electrophiles such as activated esters [39] , sulfonyl chlorides [13] or isothiocyanates [40] . Indeed, Edman degradation, the classical reaction of N-terminal protein sequencing, relies on N-terminal modification with phenyl-isothiocyanates. Unsaturated aldehyde esters are also finding increasing favour due to their ability to undergo selective irreversible azo-electrocyclizations, such as in the installation of positron-emitting-metal-binding ligands [41] . An alternative, well-established reaction for modification at lysine residues is through reductive alkylation using aldehydes in the presence of sodium cyanoborohydride [42] . The higher stability of this reagent over sodium borohydride allows selective reaction at an appropriate pH, although the rates of reaction may be sluggish due to slow imine/iminium formation in water. Iridium catalysis utilising formate as reductant can accelerate the reaction [43] . While lysine is typically the most nucleophilic amine in proteins, the N -terminus may display unique reactivity. N-terminal modification in the seminal coupling of a N-terminal cysteine and a C-terminal thioester via the ‘native chemical ligation’ (NCL) reaction is one of the most important methods for the synthetic construction of the backbone of polypeptides. Since its introduction by Kent [8] , [44] , NCL has been used extensively for the generation of synthetic proteins [45] . The intermolecular formation of an intermediate thioester is followed by a rapid S→N-acyl shift [46] , resulting in the formation of native peptide bond. Applications in fully synthetic proteins have been reviewed elsewhere [45] , [47] and many amino acids can now be generated at the ligation site in place of cysteine [48] . NCL may also be utilized in the ‘semi-synthesis’ or ‘expressed protein ligation’ of proteins through the site-selective ligation of recombinantly derived thioesters and synthetic peptides [49] . In these latter methods thioesters are usually generated by exploiting the protein self-splicing activity of inteins [50] , [51] . Recent work by Vila-Perelló et al . [52] has greatly improved the generation and purification of recombinant thioesters, allowing the semi-synthesis of proteins to gain increasing utility as a method for protein modification. The NCL reaction is perhaps illustrative of the features of success in protein chemistry since it relies in essence on enhanced, synergistic chemoselectivity derived from more than one functional group in combination (proximal amine and thiol, see Box 2 ). The reaction of an N-terminal Cys with cyanobenzothiazole, which ‘borrows’ from the chemoselectivity in the last step of luciferin formation, can be viewed similarly [53] . The N -terminus has also been used to generate uniquely reactive ketones via biomimetic transamination mediated by the co-factor pyridoxal-5′-phosphate (PLP; see section entitled Manipulating carbonyls to C protein =N bonds). The different p K a of the N -terminus can also be used to exploit pH-dependent chemistry with resulting differences in reactivity and selectivity. Box 2: Comparing strategies for positional control. Site-selective conjugation techniques take place with exquisite control of chemo- and regioselectivity. While most conjugation techniques rely on unique chemical reactivity, others may rely on, or are influenced by, the positioning of amino-acid side chains to drive selectivity. For example, thioester-mediated native chemical ligation relies on functional group proximity to generate a specificity of ligation [44] . The key spontaneous S→N-acyl shift is promoted by the favourable geometric orientation of the amine and thioester, based on the principles first reported by Wieland et al . [46] Without this proximity effect, any amine or thiol could in principle react to give a mixture of polypeptide products. Other examples of positional control include the use of short peptide sequences, which bring reactive amino acids into close proximity, leading to enhanced binding. This has been elegantly demonstrated by the group of Tsien, who have utilized the affinity of a tetra-cysteine motif, in the correct orientation to strongly bind a range of organic arsenicals. The fluorescein arsenical helix binder, or FLAsH, tag system has been of particular use due to its use in the florescent labelling of proteins, based on a minimally disrupting short amino-acid sequence [191] , [192] . Recently, the group of Hamachi has developed a novel solution to the problem of using ligand-directed conjugations to modify enzymes, namely, that the presence of the ligand usually renders the enzyme inactive. By using a ligand-directed, S N 2 reactive, tosyl group bound to the probe of interest, the ligand is released on conjugation and so does not compromise protein function [193] . The amino acids modified by this technique include non-traditional nucleophilic amino acids such as histidine and glutamic acid, strongly suggesting this as a reaction driven by proximity, rather than nucleophilicity [194] . These examples illustrate importantly that while analyses based on functional groups alone are strategically useful, they are just one aspect. Chemistry, at its best, is a sophisticated science that is not best-served by a ‘building-block-like’ approach only. Analysis of context and substrate complexity are likely to be vital tools in Chemical Biology. UAAs present an immediately obvious opportunity to provide potentially unique chemical handles at which to undertake site-selective modification of proteins in a more broad and free-ranging way than at natural. Yet, modification of such residues can be limited by methods for their installation and the chemistry available for reaction. Here we try to give illustrative examples of both and aim to do so in a representative manner. Yet, it should be noted that many hybrid strategies that ultimately exploit the same functional groups and bond-forming processes can be considered in other ways, which are not exhaustively discussed here, such as through the use, for example, of chemoenzymatic methods to first perform an enzymatic attachment of a functional group or ‘tag’ that is then reacted. Staudinger amide N protein –C bonds The Staudinger ligation between an azide and triarylphosphine, an extension of the Staudinger reaction [54] , was a conceptually exciting development. Here, elegantly, an electrophilic trap was used to divert hydrolysis of the intermediate aza–ylid, generating instead a stable amide bond ( Fig. 3a ) [55] . This has allowed the modification of azido-glycoproteins incorporated into the cell-surface glycocalyx of eukaryotic cells via the sialic acid biosynthetic and metabolic machinery. Indeed, the modification of sugars in glycoproteins was subsequently shown to be applicable to the remodelling of cell surfaces in living animals, demonstrating an apparently good level of biocompatability [5] . With the development of techniques for site-specifically incorporating azido-amino acids, this ligation became applicable to the direct modification of protein side chains, first at auxotroph-incorporated azidohomoalanine [56] and subsequently at 4-azidophenylalanine incorporated by amber-stop codon suppression [57] (see Box 3 ). Applications of Staudinger ligation in bioconjugation have been reviewed [58] , with uses as diverse as fluorogenic labelling [59] , epitope tagging of G-protein-coupled receptors [60] and the installation of photoswitches [61] . 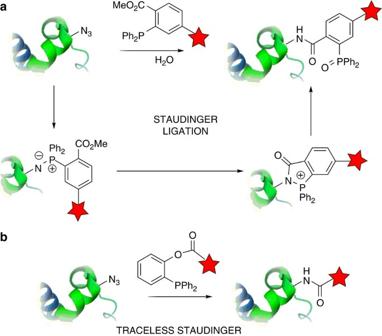Figure 3: The Staudinger ligation. (a) A ‘bio-orthogonal’ labelling of protein azides55. (b) ‘Traceless’ Staudinger variants involve loss of the phosphorus-containing prosthetic group63. Figure 3: The Staudinger ligation. ( a ) A ‘bio-orthogonal’ labelling of protein azides [55] . ( b ) ‘Traceless’ Staudinger variants involve loss of the phosphorus-containing prosthetic group [63] . Full size image Soon after the initial report, a ‘traceless’ variant was reported by the groups of Raines [62] and Bertozzi [63] . Thus, an amide bond can be generated without residual phosphine oxide ( Fig. 3b ). Other variants such as a three-component Staudinger ligation have allowed the site-specific installation of amide-bonded glycomimetics [64] , [65] . More recently, Serwa et al . [66] reported a phosphite-Staudinger reaction with a stalled intermediate phosphoramidate. In addition to negating the problem of possible phosphine oxidation [67] , this ‘traceless’ reaction valuably allows installation of phosphate mimics [66] . Despite its obvious strengths, the use of the Staudinger ligation has diminished recently due to slower associated kinetics, the retained triarylphosphine oxide appendage in ‘non-traceless’ variants and problems related to phosphine oxidation and possible side reactions of phosphines in ‘traceless’ variations [65] , [67] . Box 3: Incorporation of unnatural amino acids into proteins. The modification potential of native proteins is typically restricted by the limited functionalities afforded by the 20 canonical amino acids, particularly when multiple residues are present in a protein. Much work has therefore focused on manipulating the genetic machinery of cells to incorporate unnatural amino acids (UAAs). Often these methods rely on the reassignment of codons to a given UAA. The oldest methods for UAA incorporation utilize auxotrophic strains for a particular amino acid. Such strains cannot biosynthesize the amino acid and require uptake from the growth media [2] . The flexibility of tRNA synthetases can then be exploited to replace the natural amino acid with a structurally similar analogue. This has most commonly been utilized to incorporate azide- and alkyne-containing amino acids into methionine auxotrophic E. coli strains [56] . While many amino acids have been successfully incorporated by such a method, this reassignment of sense codons results in global incorporation of the amino acid, limiting uses in vivo and sometimes leading to cellular toxicity at higher concentrations. An alternative approach utilizes the reassignment of stop (nonsense) codons, such as the amber codon UAG, to incorporate a UAA [195] . The technique can be made to rely on an orthogonal suppressor tRNA/tRNA synthetase (tRNA/aaRS) pair, capable not only of charging the desired amino acid to a tRNA specific for the codon, but also effectively invisible to any of the endogenous cellular tRNA machinery. This has most commonly been achieved by transferring a tRNA/aaRS from another kingdom into the organism of interest, and has been achieved in both prokaryotic [195] and eukaryotic cells [151] . The two most commonly used systems are based on the tyrosine tRNA/aaRS from the archaebacteria Methanococcus jannaschii and the pyrrolysine tRNA/aaRS of Methanosarcina barkeri/mazei [196] . These pairs have been used to incorporate an incredibly diverse range of over 150 UAAs possessing varied structures, functionalities and reactive handles. This technique benefits from allowing the incorporation of a UAA at a single site of a single protein within a cell, allowing for an unprecedented degree of site selectivity. Among the UAAs incorporated by such methods are the key reactive handles for all the reactions discussed in this review. Yet, limitations of the technology remain: most importantly these include the need for more widespread access to the required plasmids and the global applicability towards all protein systems. However, recent impressive advances in the field such as amber suppression in living animals [197] , [198] , and significant increases in suppression efficiency by knockout of the gene for RF1 in E. coli [199] are beginning to open up the possibility of amber-stop codon suppression becoming an indispensable tool for the incorporation of unnatural ‘tags’ into proteins to undertake site-selective modification. The creation of an ‘amber-free’ E. coli variant is also farsighted in this regard [200] . Unnatural amino acids. A selection of unnatural amino acids that can be incorporated site selectively into proteins via reassignment of sense or nonsense codons and that could be used as ‘tags’ for the reactions discussed in this review. Heterocycles from formal or concerted cycloadditions In 2002, the groups of Sharpless [68] and Meldal [69] independently reported a stepwise modification of a classical reaction of organic chemistry, the Huisgen [70] –Dimroth [71] –Michael [72] 1,3-dipolar-cycloaddition between an azide and alkyne. They found that triazole formation was dramatically accelerated by the use of copper(I) even at room temperature, and was highly tolerant of both water and oxygen ( Fig. 4a ). The reaction was rapidly embraced by those seeking a more modular and less bespoke approach to molecular additions and has since found widespread use in the pharmaceutical and material industries, but its impact on bioconjugation has been particularly telling, initiating a number of formal and actual cycloadditions that have expanded the ability to label biological systems [73] . 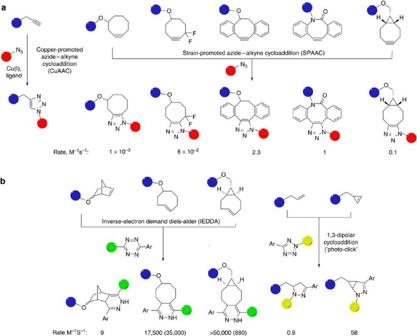Figure 4: Reactive handles used for formal and actual cycloadditions on proteins. (a) CuAAC68and SPAAC90, and (b) IEDDA101and ‘photo-click’112reactions for site-selective protein modification with reported rates for small-molecule models (‘on-protein’ rates are given in brackets where reported). No rate is given for CuAAC due to the additional dependence on copper concentration. Figure 4: Reactive handles used for formal and actual cycloadditions on proteins. ( a ) CuAAC [68] and SPAAC [90] , and ( b ) IEDDA [101] and ‘photo-click’ [112] reactions for site-selective protein modification with reported rates for small-molecule models (‘on-protein’ rates are given in brackets where reported). No rate is given for CuAAC due to the additional dependence on copper concentration. Full size image The absence and reasonable inertness of azides and alkynes in biology has made the copper-catalysed azide–alkyne ‘cycloaddition’ (CuAAC) an excellent candidate for undertaking modification of biomolecules (although it should be noted that the CuAAC is not a true cycloaddition, rather proceeding via a metallocyclic intermediate [74] ). In early demonstrations, Wang et al . [75] coated cowpea mosaic virus with azide or alkyne moieties via nonspecific lysine labelling and then undertook CuAAC reactions to fluorescently label the capsid. Despite some limitations, such as need for organic co-solvent, unspecific labelling, incomplete conversions and breakdown in capsid structure, the selectivity of triazole formation gave a major indication of the potential power of the reaction. Soon after Speers et al . [76] reported that CuAAC could be undertaken highly selectively in cellular lysates for activity-based profiling of intracellularly labelled proteins, thereby demonstrating potential tolerance towards cellular components. As with the Staudinger ligation, the ability to site-specifically incorporate UAAs into proteins allowed expanded application of the CuAAC. Having previously reported the incorporation of azide- and alkyne-containing UAAs into proteins in Escherichia coli via amber-stop codon suppression, the group of Schultz [77] reported the incorporation of both O -propargyltyrosine and p -azidophenylalanine into proteins in Saccharomyces cerevisiae . They went on to demonstrate selective labelling of these UAAs using CuSO 4 and copper wire (as indirect sources of Cu(I)) at 37 °C. Despite only partial conversions, these examples represented the first site-specific CuAAC on protein surfaces. In a series of papers, the group of Tirrell [78] , [79] , [80] reported that azide-containing amino acids could act as substrate surrogates for E. coli methionyl transfer RNA (tRNA) synthetase, resulting in their incorporation into cellular proteins. It was demonstrated that these ‘tagged’ proteins could undergo CuAAC to label the cell surface of E. coli for the first time [78] , [79] , as well as be used to identify newly synthesized proteins from stable cell line lysates [80] . This work importantly identified copper(I) bromide as a more efficient source of Cu(I) negating the need for an added reductant, yet a cellular toxicity of the metal catalyst to E. coli was suggested, with some exposed cells showing an unusual phenotype [78] , [81] . Although not yet precisely delineated, this toxicity has been attributed to the generation of reactive oxygen species that may cause intracellular damage [82] , implying that control of the Cu(I) oxidation state may prove key to effective reactions. Perhaps at odds with a notion of general toxicity is the fact that several essential proteins in organisms utilize copper, leading in some cases to a relatively high cellular content [83] . For example, in yeast, estimates of over 10 5 atoms per cell have been made with a relatively low associated toxicity as judged by MIC 50 of >0.7 mM [84] . Lack of toxicity is attributed to a highly conserved biological system for maintaining Cu(I) bound to a series of carriers, preventing the release of free copper ions that could generate reactive oxygen species. Therefore, ligands such as THPTA [83] , BTTES [85] and histidine [82] that have been used to generate Cu(I) complexes and that maintain and stabilize the metal oxidation state while also negating the potential toxicity of exogenous reductants seem a logical approach. Indeed, these have allowed the labelling of living systems including the labelling of glycans in developing zebrafish embryos [85] . Moreover, an alternative approach has recently been reported by Uttamapinant et al . Rather than reducing the toxicity of the catalyst, they used chelating azides, leading to a significant reduction in the required metal loading; this too allowed cell-compatible labelling [86] . Despite these developments, the use of CuAAC for intracellular modification in live cells is still to be reported and it is worth considering that eukaryotic cells are likely to offer additional unique challenges, which may be highly dependent on cell type. Despite possible cellular limitations, CuAAC remains invaluable for in vitro protein modification, due to its high specificity, reasonably fast reaction rate and ease-of-use. This has led to a wide range of CuAAC reagents now being commercially available for bioconjugation. Indeed, the CuAAC can be performed site-selectively with complete conversion [34] and has been used in many significant applications, such as the generation of PEGylated proteins [87] , the generation of dual PTM glycoprotein mimics due to its orthogonality to existing cysteine chemistry [34] , [35] , cellular proteomic analysis (BONCAT) [80] , a quantitative method for primary cell proteomics (QuaNCAT) [88] , and the construction of highly-valent protein nanoparticles [89] . Despite this compatibility, the perceived toxicity of copper has led to the exploration of alternative cycloaddition-type reactions. The group of Bertozzi [90] has removed copper from the equation entirely, first reporting a strain-promoted azide–alkyne cycloaddition (SPAAC) in 2004. Building on work by Wittig and Krebs [91] in the 1960s, they found that highly strained cyclooctynes reacted rapidly at room temperature with azide-‘tagged’ glycoproteins in a reaction requiring no exogenous ligands or catalysts. No toxicity was observed during the reaction on the surface of mammalian cells. In its original format, the SPAAC reaction displayed similar, relatively slow, kinetics to the Staudinger ligation ( Fig. 4a ) [67] . To improve the rate, both difluorinated cyclooctynes [92] (DIFO) and dibenzocylooctynes [93] were independently reported allowing the visualisation of dynamic processes. In a particularly striking example, Laughlin et al . [94] utilized DIFOs to visualize the development of glycans during zebrafish embryo growth, demonstrating a high degree of specificity and ‘bio-orthogonality’ at slightly faster rates than previously reported using the Staudinger ligation. Further enhancements in rates have been reported through the generation of biarylazacyclooctynones [95] and cyclopropyl-fused bicyclononynes [96] ( Fig. 4a ). The site-specific incorporation of cyclooctynes [97] and biscyclononynes [98] into proteins by amber-stop codon suppression has also recently been reported. However, limitations remain, such as occasional difficulty in the synthesis and handling of strained and unstable compounds, while crucially a degree of incompatibility towards cysteine has been reported [99] , [100] . In addition, these reactions remain relatively slow ( Fig. 4a ). As a general comment, many reported rate constants used to compare protein reactions have typically been calculated under conditions that often vary significantly, and most in fact not even on proteins but on small-molecule models; thus, direct comparison of rates should be undertaken with some caution and different derivatives may be more applicable to certain situations than others. Inspired by the development of SPAAC reactions, the groups of Fox [101] and Hilderbrand [102] began to investigate the use of inverse-electron demand Diels-Alder (IEDDA) reactions as a method for bioconjugation. It was found that the reactive dienes trans -cyclooctene [101] and norbornene [102] react relatively rapidly with suitable tetrazine dienophiles (which release nitrogen irreversibly on subsequent retro-[4+2]-cycloaddition) allowing protein labelling at rates up to 1,000 times faster than SPAAC in the case of trans -cyclooctene ( Fig. 4b ). Inspired by the work of Dommerholt et al . [96] , it was found that trans -bicyclononene reacted at yet faster rates (while noting the caveats on rate determinations given above) [103] . In addition to allowing labelling of highly dynamic processes, such rapid and efficient reactions allow the concentrations of reactive partners to be lowered significantly, reducing background labelling particularly in cases where it is implausible to wash away excess reagent, such as intracellularly or in animal models [104] . To generally enable IEDDA protein reactions, key reactive UAAs (tetrazine [105] , norbornene [106] , [107] , [108] , cyclooctene [98] , [107] and biscyclononene [98] ) have been incorporated into proteins by amber-stop codon suppression (see Box 2 ). Such strain-promoted cycloadditions offer intriguing and exciting possibilities for future protein labelling where the speed of labelling is vital, and recent developments suggest that the cyclooctyne-azide and cyclooctene-tetrazine reactions may have a degree of mutual compatibility, thereby allowing multi-site labelling [109] , [110] . Some limitations remain, such as the isomerisation of trans -cyclooctenes in the presence of thiols [98] (cf reaction of thiols with cyclooctynes noted above) and the potential instability of tetrazines [110] . Also, in many variants of these SPAAC and IEDDA, reaction mixtures of regioisomers are formed (unlike the CuAAC, which is highly 1,4-selective) and in some cases bulky linkages may prevent effective syntheses of functional structures (as opposed to those that have simply been labelled) such as PTM mimics, which can often be quite small and structurally subtle. An intriguing alternative approach to cycloadditions on proteins has been reported in a series of papers by Lin. Some tetrazoles can act as latent sources of nitrile imines, which can undergo [3+2]-cycloadditions with unactivated alkenes ( Fig. 4b ) [111] . Their generation requires irradiation with ultraviolet light (this is termed a ‘photo-click’). The reaction has been used to modify a number of alkenyl-UAAs site specifically, such as homoallylglycine [112] and cyclopropenes [113] , while the genetic incorporation of tetrazoles has also been achieved as a reactive handle for undertaking ‘photo-click’ reactions [114] . While the rates of reaction are now approaching levels seen for norbornene–tetrazine conjugations, the reaction is still somewhat slower than cyclooctene–tetrazine reactions. Nonetheless, the ability to spatially and temporally control the reaction through light makes the ‘photo-click’ an attractive alternative for the site-specific labelling of proteins [113] . Metal-mediated C protein –C or C protein =C bonds Transition metal (TM) catalysis has revolutionized organic synthesis with the ability to tune reactivity by careful choice of metal, ligand and reaction conditions, allowing the generation of previously inaccessible carbon and heteroatom-containing scaffolds. Many of the factors that make such reactions appealing to the synthetic chemist also make them attractive for protein modification [115] . Such reactions are often associated with excellent functional group tolerance and high yields under mild conditions, while the reactive handles utilized are often inert in biological systems. However, restrictions such as a need to proceed efficiently at low protein loadings, solely in aqueous media, and to tolerate potential nonspecific binding to the multitude of possible Lewis-basic residues on protein surfaces, until recently, hindered the use of such reactions for site-specific protein modification. Arguably, the most widely used TM-catalysed reactions in organic synthesis are the series of palladium-catalysed sp 2 –sp 2 coupling reactions between aryl/alkenyl halides and a variety of coupling partners such as boronic acids (Suzuki–Miyaura), alkenes (Mizoroki–Heck) and alkynes (Sonogashira). Early examples of couplings on short synthetic peptides required high temperatures, or the presence of organic solvents, yet demonstrated tolerance of Pd towards some amino-acid functional groups [116] , [117] . Despite the UAA p -iodophenylalanine having been incorporated into proteins by amber-stop codon suppression and proposed as a Pd coupling partner as early as 2002 (ref. 118 ), it was not until 2006 that this was partially realized by Kodama et al . Both Heck and Sonagashira reactions were demonstrated, albeit in low yields (2% Heck, 25% Sonagashira), representing early examples of Pd-catalysed couplings on polypeptidic substrates [119] , [120] . Brustad et al . [121] then went on to demonstrate that p -boronophenylalanine could be used to undertake Suzuki couplings, although again low yields (30%) and high temperatures (70 °C) that caused protein denaturation limited the usefulness of the reaction. It was not until 2009 that Chalker et al . [122] demonstrated the first efficient Pd-mediated reaction on a protein, through the discovery of a water-and-air-stable ligand, 2-amino-4,6-dihydroxypyrimidine (ADHP, L1), for undertaking Suzuki–Miyaura cross-couplings at 37 °C in water at pH 8 ( Fig. 5a ). This allowed a variety of boronic acids to be coupled to a model cysteine-linked aryl iodide, with the benefit that even hydrophobic moieties could be transferred to the protein surface due to the water-solubilizing effect of the boronate group. To generalize this reaction to genetically incorporated amino acids, Spicer and Davis [123] (and later Liu et al . [124] ) demonstrated that through amber-stop codon suppression, p -iodophenylalanine could be used as a reactive handle for protein Suzuki–Miyaura cross-coupling. During this work, previously hypothesized weak, nonspecific binding of TMs to Lewis-basic amino acids was encountered under some conditions, leading to ambiguity in reaction analysis; this was circumvented by the identification of a suitable palladium scavenger. The group of Davis has since gone on to demonstrate that the Suzuki–Miyaura reaction is applicable to couplings on the cell surface of E. coli , demonstrating a negligible catalyst toxicity [125] , and that the coupling of carbohydrate–boronic acids to cell surfaces can be used to mimic glycoproteins in a cellular synthetic glycocalyx [125] , [126] . 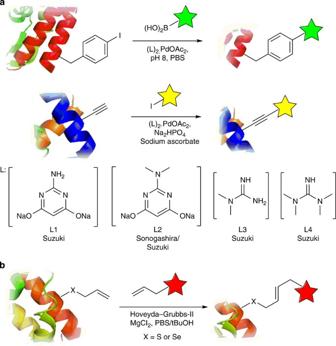Figure 5: TM-mediated protein chemistry. Use of (a) Suzuki122,123and Sonagashira couplings127, and (b) olefin metathesis,131,135for protein modification. Figure 5: TM-mediated protein chemistry. Use of ( a ) Suzuki [122] , [123] and Sonagashira couplings [127] , and ( b ) olefin metathesis, [131] , [135] for protein modification. Full size image Although ADHP is an efficient catalyst for undertaking Suzuki–Miyaura cross-couplings, it can be less effective for other Pd-catalysed reactions. Li et al . [127] have since shown that by simple methylation of the ligand, the same catalytic system could be used to promote Sonogashira reactions (L2 in Fig. 5a ), while the minimal motif guanidine-based ligands (L3 and L4 in Fig. 5a ) can significantly enhance the rate of Suzuki reactions relative to ADHP [128] and allow efficient couplings even at low stoichiometries and concentrations suitable when labelling with scarce reagents [129] . It was also shown that PEG chains offer new reactivity and a significant enhancement in rate as self-liganding (internally chelating) boronic acids when used with Pd(OAc) 2 to give a high-yielding site-specific PEGylation of proteins [128] . This self-liganded effect has more recently been exploited by Li et al . [130] , who found that PEG-conjugated fluorophores with Pd(NO 3 ) 2 could efficiently catalyse the Sonogashira cross-coupling, even intracellularly, in E. coli and Shigella . Olefin metathesis has also found recent application in the site-selective modification of proteins, due to the discovery by Lin et al . [131] that allyl sulfides are privileged substrates for undertaking aqueous cross-metathesis with Hoveyda–Grubbs II catalyst, via a proposed sulfur-relayed mechanism ( Fig. 5b ). The subsequent use of a variety of olefinic amino-acid side chains containing allylic heteroatoms suggested a breadth for this allylic chalcogen effect [132] . This allowed the installation of a number of olefin substrates including PEG and allyl glycosides at an S-allyl cysteine residue, introduced into proteins via a number of chemical routes [133] . Determination of sensitivity to accessibility, self-metathesis and reagent reactivity has delineated predictive rules for this protein reaction [134] . Moreover, tuning of heteroatom (S→Se) in Se-allylselenocysteine led to a significant increase in reaction rate and expanded substrate scope [135] ; this was applied to a chemically controlled ‘write-read-erase’ histone protein modification cycle. A further example of intriguing TM catalysis was first reported by Antos and Francis [136] , utilising rhodium-generated carbenoids formed from diazo reagents for modification of tryptophan residues. While this reaction initially required quite harsh acidic conditions (pH 3), it was subsequently found that this was primarily to denature early protein substrates and hence to expose the reactive tryptophan residue; conjugations at pH 6 are now possible [137] . Recent reports by the group of Ball [138] , [139] have used rhodium-bound metallopeptides to catalyse modification of tryptophan by using a structure-directed approach. Despite this elegantly designed rate enhancement, the need for a highly specific interaction to direct the reaction will likely limit its general applicability. However, it represents an impressive example of molecular recognition to override inherent reactivity. Given the strength and ubiquity of carbon–carbon bonds, there will be continuing utility in their formation, despite the potential of heteroatom–carbon bond-forming chemistry. We have focused in this section on metal-mediated processes since, thus far, they have dominated current strategies, yet it should be noted that other possible strategies exist that exploit non-metal-mediated processes, such as aldol [140] or Wittig chemistry [141] , the use of (formal) cycloaddition chemistry or as the result of a relay from a prior bond-forming event (for example, Pictet–Spengler). Manipulating carbonyls to C protein =N bonds Despite being widespread throughout nature, the carbonyl groups of aldehydes and ketones are almost entirely absent from native proteins [142] . Yet, the diversity of unique chemistry that they can undergo in the presence of the natural functional groups of proteins makes them an attractive handle for protein modification. They have found particular use in the reaction of hydrazines and hydroxylamines to form hydrazones and oximes, respectively, under acidic conditions (in part due to reagent availability and ease of use). These reactions can be accelerated by nucleophilic catalysts such as aniline [143] . To install aldehydes and ketones into proteins, a number of methods have been identified. Among the earliest was the discovery that periodate oxidation (cleavage) of N-terminal Ser/Thr residues led to a terminal aldehyde, which could then react selectively with a fluorescent hydrazine to allow site-specific protein tagging [144] . The group of Francis [145] has utilized a biomimetic PLP-mediated transamination to generate N-terminal ketones. Investigation of the reaction conditions indicates that a range of amino acids are tolerated by this reaction [146] , allowing the selective modification of antibodies [147] and filamentous phage [148] . The genetic incorporation of a ketone-containing amino acid by amber-stop codon suppression was first reported by Cornish et al . [149] via chemical acylation of a tRNA synthetase. This residue, once installed, again reacted selectively with a range of fluorescent hydrazines. The ketone amino acids p -acetylphenylalanine [142] and m -acetylphenylalanine [150] were subsequently incorporated into proteins, without the need for chemical acylation, in both E . coli [142] , [150] and eukaryotic cells [151] . More recently, Huang et al . [152] reported the incorporation of aliphatic ketone-containing amino acids that showed improved reaction kinetics, while diketone-containing amino acids have been reported to give increased stability in oxime products [153] . Alternatively, Carrico et al . [154] have exploited a six-residue sequence tag that directs a natural formylglycine-generating enzyme in both prokaryotic and eukaryotic cells. The subsequent formation of hydrazones and oximes from these carbonyls has found widespread use in the conjugation of functional handles and probes to proteins. For example, hydroxylamines have been used to generate glycoprotein mimics [155] , to label G-protein-coupled receptors [156] , antibodies [157] and therapeutic proteins for increased pharmacokinetics [6] , and for dual protein tagging and formation of bifunctional antibodies [158] , [159] . However, despite its widespread use, the reactions of aldehydes and ketones suffer from a number of key drawbacks. Most importantly, due to the presence of a range of carbonyl-containing substrates in cells, this chemistry is not necessarily suitable for in vivo applications. In addition, the hydrazone and oxime linkages are inherently unstable, leading to hydrolysis over the course of hours, particularly under acidic conditions, although hydroxylamines are reported to generate more stable linkages [160] . To avoid such instability, Sasaki et al . [161] recently reported the use of a modified Pictet–Spengler reaction for aldehyde modification (which ultimately leads to the subsequent creation of C–C and C–N bonds), with Agarwal et al . [162] subsequently reporting greatly improved reaction kinetics. Although the fundamental limitation of a lack of bioapplicability still remains, the facile use of aldehyde/ketone chemistry remains an attractive tool for in vitro modifications. C protein –S/Se bonds The UAA dehydroalanine (Dha) can be used as a Michael acceptor and has found extensive use in protein modification, reacting rapidly with sulfur nucleophiles to generate alkyl cysteine analogues, offering an electrophilic alternative to nucleophilic reaction of cysteine [3] . This is particularly useful in examples where use of electrophilic alkylation of Cys is difficult to control or where appropriate electrophiles cannot be generated, and leads to a greater level of selectivity. Dha can be accessed via a number of routes: elimination of active-site serines, the oxidative elimination of unnatural selenocysteine amino acids [163] , [164] or through the milder oxidative elimination of cysteine with sulfonylhydroxylamine reagents [165] . All can prove efficient but occasional side reactions in all recently prompted the development of a bis-alkylation method: cyclic sulfoniums can be eliminated to form Dha under strikingly mild conditions [166] . The addition of functionalized thiols to Dha takes place rapidly and selectively under mild conditions. This reaction has been used to install a number of thioether mimics of natural protein modifications such as lipidation, glycosylation, phosphorylation and lysine methylation/acetylation [164] , [165] , [167] , [168] , as well as installing reactive handles for further modification such as S -allyl cysteine for olefin metathesis. [131] These reactions typically (but not always) proceed with low substrate control in their diastereoselection and so a mixture of D / L -epimers is produced at the site of modification. Dha also provides a viable method for chemically creating selenocysteines in proteins [135] . Although only shown for a single example (Se-allyl cysteine), the discovery of conditions for creating suitable Se nucleophiles for this addition may enable broader methods. While the olefin in Dha displays unique conjugate electrophile reactivity, isolated olefins in, for example, homoallylglycine can serve as useful UAAs for modifications using radical chemistry (see Box 1 ) [169] . The introduction of site-directed gene mutagenesis as a powerful method for altering protein structure at a genetic level revolutionized the study and application of proteins. The ability to switch between natural amino acids at virtually any desired residue site in a recombinant protein has allowed unparalleled progress in the manipulation of proteins for scientific discovery. Yet, this ability to access and alter functionality is limited by the 20 typical proteinogenic amino acids and a limited palette of chemical functional groups. As such, there is a powerful need for chemical modification of proteins and the installation of non-natural functionality as a strategy for more free-ranging protein synthesis or design. New methods should aspire to the widespread success and applicability of gene mutagenesis as a tool in the biological sciences [12] . Over the past 15 years, the field of chemical protein modification has been dramatically revitalized, from one that focused on the use of natural cysteine and lysine residues to one that now utilizes a wide range of chemical handles, coupling partners and conditions, many of which are mutually compatible (‘orthogonal’) not just with (to) each other, thereby allowing multiple modifications to be undertaken, but also with (to) living systems, allowing them to be utilized in vivo [170] . The use of such reactions is only beginning to be exploited as improvements in selectivity, kinetics, compatibility and ease of use are made. The potential applications of modified proteins are virtually limitless, whether be it for the in vivo tracking of dynamic processes, the conjugation of therapeutic agents, the elucidation of biosynthetic/metabolic pathways or the use of modified protein-based materials with novel functionality and structure. The development of these reactions has been reviewed here from the viewpoint of applicable chemistry, rather than the biological uses of modified proteins, and it is likely that with an expanding toolkit of chemical reactions for installing a range of modifications, chemists and biologists will discover exciting applications as yet unexplored. This could truly become an unlimited form of Synthetic Biology. Since such protein methods have become a ‘hot-topic’ over the past decade, it has been easy to forget some critical principles in developing chemical reactions for modifying proteins. Sadly, increasing numbers of reports are now simply undertaking reactions ‘because one can’ with little-or-no regard for improving (either strategically or functionally) on the plethora of reactions already available. We see a particular need to develop chemical reactions that allow: the selective installation of a desired functionality in a manner that allows the mimicry of a natural modification, the rapid labelling of a biologically relevant site or new in vivo reactivity. We see less value in the discovery of those reactions that may not have been performed on a protein previously but in fact offer no benefit compared with the existing ‘toolkit’. Put more succinctly, there is not necessarily a need for new chemistry for modifying proteins; there is a need for better chemistry for modifying proteins. It is important to remember that proteins should not be seen merely as a substrate for undertaking a reaction. Rather, this chemistry should be increasingly seen as a method for testing a hypothesis, developing the technology or creating a functional probe. To this extent, a number of key challenges can be envisaged that must be addressed in future developments in the field. While the reactions discussed here represent useful discoveries that will undoubtedly make a large impact on protein science, they are not without their limitations. A reaction that combines the ‘selling points’ of each must be seen as highly desirable: the mimicry and minimal linker afforded by cysteine, the ease of modification at lysine, the bio-orthogonality of the Staudinger ligation, the unparalleled speed of cycloadditions, the tunability of transition metal-mediated reactions, the potential reversibility and switching of carbonyl chemistry. A reaction that combines these favourable characteristics may represent an ideological end goal in the development of new chemistries. When judged by these criteria of utility, protein chemistry is still in its infancy. As it matures, it will likely revolutionize the molecular analysis of Biology. How to cite this article: Spicer, C. D. and Davis, B. G. Selective chemical protein modification. Nat. Commun. 5:4740 doi: 10.1038/ncomms5740 (2014).